Impaired endolysosomal function disrupts Notch signalling in optic nerve astrocytes Astrocytes migrate from the optic nerve into the inner retina, forming a template upon which retinal vessels develop. In the Nuc1 rat, mutation in the gene encoding βA3/A1-crystallin disrupts both Notch signalling in astrocytes and formation of the astrocyte template. Here we show that loss of βA3/A1-crystallin in astrocytes does not impede Notch ligand binding or extracellular cleavages. However, it affects vacuolar-type proton ATPase (V-ATPase) activity, thereby compromising acidification of the endolysosomal compartments, leading to reduced γ-secretase-mediated processing and release of the Notch intracellular domain (NICD). Lysosomal-mediated degradation of Notch is also impaired. These defects decrease the level of NICD in the nucleus, inhibiting the expression of Notch target genes. Overexpression of βA3/A1-crystallin in those same astrocytes restored V-ATPase activity and normal endolysosomal acidification, thereby increasing the levels of γ-secretase to facilitate optimal Notch signalling. We postulate that βA3/A1-crystallin is essential for normal endolysosomal acidification, and thereby, normal activation of Notch signalling in astrocytes. Notch signalling is involved in numerous functions including pattern formation during development and gliogenesis [1] , [2] . The Notch pathway is evolutionarily conserved and promotes the generation of astrocytes from neuronal precursor cells [3] , [4] . Four Notch receptors, Notch1–4, have been identified. The Notch gene encodes a single-pass transmembrane protein, which appears on the cell surface as a heterodimeric protein after maturing along the secretory pathway [5] . Notch receptors are activated by interaction with transmembrane ligands expressed on the surface of juxtaposed cells. Binding of the ligands activates two sets of proteolytic cleavages in the Notch receptor. First, TNFα-converting enzyme, a member of the ADAM family of matrix metalloproteases, cleaves the receptor at its extracellular domain, generating a membrane-tethered Notch receptor [5] . Next, the receptor is cleaved within its transmembrane domain by the γ-secretase multiprotein complex (including presenilin, nicastrin, APH1 and PEN2) (ref. 6 ), resulting in release of the Notch intracellular domain (NICD); NICD translocates to the nucleus to activate Notch target genes [7] . The activation of Notch requires processing, endocytosis and trafficking of both Notch receptor and ligand. Ubiquitination has an important role in the activation of Notch signalling [8] . In recent years, it has also been suggested that endocytosis of Notch is important for ligand-mediated activation [9] , [10] . There is now a general consensus that γ-secretase-mediated S3 cleavage of Notch can occur at multiple steps within the endolysosomal compartments [11] . Increasing evidence suggests that endocytosis is involved in the transport of ligand–receptor complexes to acidic endolysosomal compartments, where low pH is required for signalling [10] , [12] . The acidic luminal environment of endosomes, lysosomes and secretory vesicles is established by the vacuolar-type proton ATPase (V-ATPase), which pumps protons into the lumen [13] , [14] , [15] . V-ATPase-dependent acidification is required to optimally activate γ-secretase, an acid protease that mediates S3 cleavage of Notch [15] . Therefore, progressive acidification of the endolysosomal system could influence the levels of NICD production. In Drosophila, various mutants that show impaired acidification due to alteration of V-ATPase activity affect Notch signalling [13] , [15] . In the past decade, several laboratories have shown that crystallins, the major structural proteins of the lens, are expressed outside of the lens and have cellular functions [16] , [17] , [18] . We previously postulated that βA3/A1-crystallin may regulate the process of programmed cell death in the developing retina and that it also has a pivotal role in maintaining the proper number of astrocytes in the retina through an anoikis-mediated cell death process [19] , [20] . We show here that βA3/A1-crystallin affects Notch signalling in astrocytes by regulating endolysosomal function in astrocytes by modulating the activity of V-ATPase. In the absence of βA3/A1-crystallin, V-APTase activity decreases and acidification of endolysosomal compartments is impaired. The higher pH inhibits the γ-secretase-mediated formation of NICD, leading to decreased Notch signalling. Optic nerve astrocytes express both Notch1 and Jagged1 Notch signalling has an important role during differentiation and maturation of the brain astrocytes [21] , [22] ; however, its role in optic nerve astrocytes is unexplored. Disrupted Notch signalling affects pattern formation in other systems [23] . We have shown major defects in template formation and honeycomb patterning by Nuc1 retinal astrocytes with mutated βA3/A1-crystallin [24] , [25] . We first studied expression of Notch pathway components in optic nerve astrocytes cultured from 2- to 3-day-old WT (wild type) and Nuc1 rats. Quantitative reverse transcriptase PCR (qRT–PCR) analysis showed that WT cells strongly express Notch1 receptor transcript ( Fig. 1a ). Nuc1 cells have 2-fold higher expression of Notch1 than WT cells. The canonical Notch ligands are single-pass transmembrane proteins belonging to the Delta-like or serrate families. Using specific primers, we tested their expression in WT and Nuc1 astrocytes. Our results show, for the first time, that optic nerve astrocytes express Jagged1 ( Fig. 1b ), with no significant expression of the Delta-like ligands. Co-localization of Jagged1 with the astrocyte marker, glial fibrillary acidic protein (GFAP), in retinal flatmounts confirms expression of Jagged1 in retinal astrocytes ( Fig. 1d ). 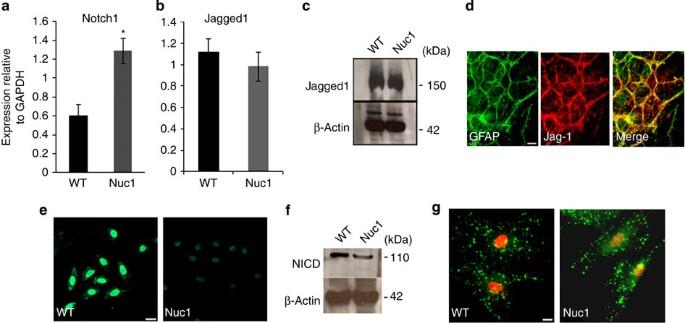Figure 1: Levels of Notch1 and Jagged1 in postnatal day 2 WT and Nuc1 optic nerve astrocytes. (a,b) qRT–PCR using Taqman expression probes shows that Notch1 was elevated by >2-fold in Nuc1 astrocytes (*P=0.027), relative to WT astrocytes. WT and Nuc1 astrocytes had similar levels of Jagged1. (c) Western analysis for Jagged1 shows similar protein levels in WT and Nuc1 astrocytes. (d) Retinal flat mounts from a 3-day-old WT rat showing significant co-localization (yellow) of Jagged1 (red) with GFAP-positive astrocytes (green). (e,f) Immunostaining and western analysis for active Notch (NICD) using anti-V1744 antibody shows that NICD was decreased by 76% in Nuc1 astrocytes compared with WT astrocytes (*P=0.0031). (g) Expression and distribution of NICD and Jagged1 as revealed by immunostaining with anti-V1744 active Notch (red) and anti-Jagged1 antibodies (green). Decreased nuclear staining for NICD was evident in Nuc1 cells, but Jagged1 staining was similar in WT and Nuc1 astrocytes. Scale bar, 20 μm. In all panels, graphs show mean values and error bars represent s.d. from a triplicate experiment representative of at least three independent experiments. Statistical analysis was performed by a two-tailed Student’st-test: *P<0.05. Figure 1: Levels of Notch1 and Jagged1 in postnatal day 2 WT and Nuc1 optic nerve astrocytes. ( a , b ) qRT–PCR using Taqman expression probes shows that Notch1 was elevated by >2-fold in Nuc1 astrocytes (* P =0.027), relative to WT astrocytes. WT and Nuc1 astrocytes had similar levels of Jagged1. ( c ) Western analysis for Jagged1 shows similar protein levels in WT and Nuc1 astrocytes. ( d ) Retinal flat mounts from a 3-day-old WT rat showing significant co-localization (yellow) of Jagged1 (red) with GFAP-positive astrocytes (green). ( e , f ) Immunostaining and western analysis for active Notch (NICD) using anti-V1744 antibody shows that NICD was decreased by 76% in Nuc1 astrocytes compared with WT astrocytes (* P =0.0031). ( g ) Expression and distribution of NICD and Jagged1 as revealed by immunostaining with anti-V1744 active Notch (red) and anti-Jagged1 antibodies (green). Decreased nuclear staining for NICD was evident in Nuc1 cells, but Jagged1 staining was similar in WT and Nuc1 astrocytes. Scale bar, 20 μm. In all panels, graphs show mean values and error bars represent s.d. from a triplicate experiment representative of at least three independent experiments. Statistical analysis was performed by a two-tailed Student’s t -test: * P <0.05. Full size image Next, we investigated the expression of NICD using anti-Notch V1744, an antibody specific for NICD. Immunostaining and western blotting detected a significant decrease in NICD protein in Nuc1 astrocytes compared with WT ( Fig. 1e ). Confocal microscopy ( Fig. 1g ) demonstrated that NICD (red) staining was primarily nuclear and weaker in Nuc1 astrocytes compared with WT, while Jagged1 (green) staining was similar in both cell types. Notch signalling is reduced in Nuc1 astrocytes As our data indicate downregulation of NICD in Nuc1 astrocytes, we examined activation of the Notch pathway using a Notch luciferase reporter assay. Notch1 receptor constructs, including a full-length receptor (Notch-FL) and truncated or mutant derivatives with varying activation profiles, were used. A constitutively active Notch construct, NδE, activates the Notch pathway in a ligand-independent manner, and the NICD construct contains only the NICD. WT and Nuc1 astrocytes were co-transfected with Notch-FL, NδE or NICD constructs, along with the 6XCBF1-luciferase Notch reporter plasmid, and the phRL-SV40 Renilla luciferase reporter plasmid. WT astrocytes, transfected with the Notch-FL construct, showed 4-fold increased activity compared with astrocytes transfected with vector only ( Fig. 2a ). Nuc1 astrocytes, in contrast, showed only minimal activation ( Fig. 2b ). The Notch pathway was activated equally in WT and Nuc1 astrocytes expressing the constitutively active NδE construct ( Fig. 2a ). Notch1 in WT astrocytes was strongly activated (~65% increase in luciferase activity compared with untreated cells) by EDTA, a Ca 2+ -chelating agent that activates Notch in a ligand-independent manner [26] . This activation was inhibited by N-[N-(3, 5-difluorophenacetyl)-L-alanyl]- S -phenylglycine t -butyl ester (DAPT), an inhibitor of γ-secretase ( Fig. 2a ). Nuc1 astrocytes, however, showed only modest activation of the Notch pathway by EDTA, although DAPT did inhibit this Notch activation ( Fig. 2b ). EDTA did not significantly influence Notch activity in either WT or Nuc1 astrocytes expressing NδE, although DAPT still was inhibitory ( Fig. 2a ). Dimethylsulphoxide (vehicle for DAPT) did not affect Notch activity in WT or Nuc1 astrocytes. 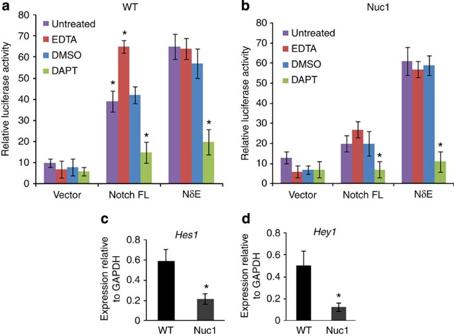Figure 2: 6XCBF-1 luciferase activity in WT and Nuc1 astrocytes transfected with Notch. (a) In WT astrocytes transfected with the Notch-FL plasmid, luciferase activity in untreated astrocytes was significantly higher (4-fold increase) than in untreated vector-transfected astrocytes (*P=0.016). Significant induction of luciferase activity was observed in the presence of EDTA in WT astrocytes expressing Notch-FL plasmid (*P=0.031), while luciferase activity was significantly reduced in the presence of the γ-secretase inhibitor, DAPT (*P=0.009) compared with untreated astrocytes. Dimethylsulphoxide (DMSO; vehicle for DAPT) alone did not affect expression significantly. Luciferase activity in WT astrocytes expressing the NδE construct was not increased by EDTA, but existing activity was inhibited by DAPT (*P=0.012). Vector-transfected cells showed basal levels of luciferase activity. (b) In Nuc1 astrocytes, transfected with the Notch-FL plasmid, there was no significant induction of luciferase activity in the presence of EDTA. Luciferase activity was significantly reduced in the presence of DAPT (*P=0.025) compared with untreated cells. Luciferase activity in Nuc1 astrocytes expressing NδE was not induced in the presence of EDTA but could be inhibited in the presence of DAPT(*P=0.007). Vector-transfected cells showed basal levels of luciferase activity. (c,d) qRT–PCR analysis for expression ofHes1andHey1in WT and Nuc1 astrocytes. Nuc1 astrocytes showed about 65 and 75% reduction in the levels ofHes1andHey1, respectively, compared with WT astrocytes (*P=0.030 and *P=0.027, respectively). In all panels, graphs show mean values and error bars represent s.d. from a triplicate experiment representative of at least three independent experiments. Statistical analysis was performed by a two-tailed Student’st-test: *P<0.05. Figure 2: 6XCBF-1 luciferase activity in WT and Nuc1 astrocytes transfected with Notch. ( a ) In WT astrocytes transfected with the Notch-FL plasmid, luciferase activity in untreated astrocytes was significantly higher (4-fold increase) than in untreated vector-transfected astrocytes (* P =0.016). Significant induction of luciferase activity was observed in the presence of EDTA in WT astrocytes expressing Notch-FL plasmid (* P =0.031), while luciferase activity was significantly reduced in the presence of the γ-secretase inhibitor, DAPT (* P =0.009) compared with untreated astrocytes. Dimethylsulphoxide (DMSO; vehicle for DAPT) alone did not affect expression significantly. Luciferase activity in WT astrocytes expressing the NδE construct was not increased by EDTA, but existing activity was inhibited by DAPT (* P =0.012). Vector-transfected cells showed basal levels of luciferase activity. ( b ) In Nuc1 astrocytes, transfected with the Notch-FL plasmid, there was no significant induction of luciferase activity in the presence of EDTA. Luciferase activity was significantly reduced in the presence of DAPT (* P =0.025) compared with untreated cells. Luciferase activity in Nuc1 astrocytes expressing NδE was not induced in the presence of EDTA but could be inhibited in the presence of DAPT(* P =0.007). Vector-transfected cells showed basal levels of luciferase activity. ( c , d ) qRT–PCR analysis for expression of Hes1 and Hey1 in WT and Nuc1 astrocytes. Nuc1 astrocytes showed about 65 and 75% reduction in the levels of Hes1 and Hey1 , respectively, compared with WT astrocytes (* P =0.030 and * P =0.027, respectively). In all panels, graphs show mean values and error bars represent s.d. from a triplicate experiment representative of at least three independent experiments. Statistical analysis was performed by a two-tailed Student’s t -test: * P <0.05. Full size image We also assessed the expression of Notch target genes using qRT–PCR. Expression of Hes1 and Hey1 was reduced ~65% and ~75%, respectively, in Nuc1 astrocytes compared with WT astrocytes ( Fig. 2c ). Jagged1 is an agonist of Notch signalling in astrocytes Our studies have shown that optic nerve astrocytes strongly express Jagged1. Previous studies have shown that Jagged1 acts as an inhibitor of the Notch signalling pathway by competitively inhibiting binding of Delta-like ligands to the Notch receptor [27] , [28] . Therefore, we sought to determine whether Jagged1 acts as agonist or antagonist in astrocytes. WT and Nuc1 astrocytes were treated with Jagged1 short interfering RNA, and Notch pathway activity was monitored by measuring expression of Hey1 and Hes1 . siRNA knockdown of Jagged1 ( Fig. 3a ) resulted in concomitant reductions in Hes1 and Hey1 , in both WT and Nuc1 astrocytes ( Fig. 3b ). 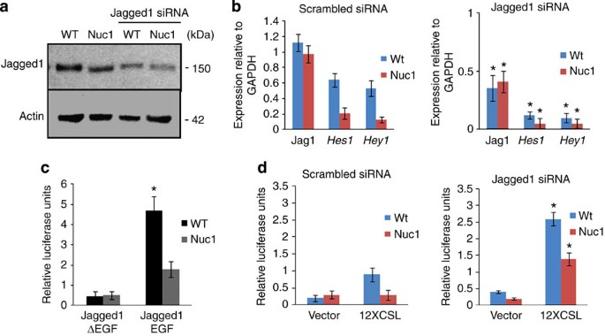Figure 3: Effect of Jagged1 on Notch signalling in WT and Nuc1 astrocytes. (a) Western analysis for Jagged1 in WT and Nuc1 astrocytes transfected with scrambled or ON-TARGET plus Smart pool Jagged1 siRNA. Downregulation of Jagged1 expression was observed in both WT and Nuc1 astrocytes transfected with the targeted siRNA. (b) qRT–PCR for the Notch pathway targetsHes1andHey1in WT and Nuc1 astrocytes after treatment with scrambled or Jagged1 siRNA. Knockdown of Jagged1 expression (*P=0.013 in WT and *P=0.017 in Nuc1) is reflected by decreased expression ofHes1(*P=0.022 in WT and *P=0.015 in Nuc1) andHey1(right panel: values relative to scrambled siRNA in left panel). (c) 12XCSL-luciferase reporter activity in cocultures of Notch1-expressing astrocytes carrying 12XCSL-luciferase reporter construct (ΔEGF) or pRL-cmv control (EGF) construct, with astrocytes overexpressing the Jagged1 ligand. Graph shows luciferase activity (arithmetic mean) from triplicates of each coculture. Robust luciferase activity was seen in WT astrocytes (*P=0.011), compared with Nuc1 astrocytes. This increase is compromised in astrocytes expressing the Jagged1 ΔEGF Notch-binding-deficient plasmid. (d) 12XCSL-luciferase reporter activity in cocultures of Jagged1 knockdown astrocytes expressing 12XCSL-luciferase reporter construct or pRL-cmv control constructs with astrocytes overexpressing Jagged1. A marked induction of Notch signalling was observed in both WT (*P=0.019) and Nuc1 astrocytes transfected with Jagged1 siRNA (*P=0.027) and cocultured with astrocytes overexpressing Jagged1 compared with scrambled siRNA-treated cells (left panel). Astrocytes transfected with empty vector were also cocultured with Jagged1 overexpressing cells, showing a modest induction of the Notch pathway in WT and none in Nuc1 homozygous astrocytes. In all panels, graphs show mean values and error bars represent s.d. from a triplicate experiment representative of at least three independent experiments. Statistical analysis was performed by a two-tailed Student’st-test: *P<0.05. Figure 3: Effect of Jagged1 on Notch signalling in WT and Nuc1 astrocytes. ( a ) Western analysis for Jagged1 in WT and Nuc1 astrocytes transfected with scrambled or ON-TARGET plus Smart pool Jagged1 siRNA. Downregulation of Jagged1 expression was observed in both WT and Nuc1 astrocytes transfected with the targeted siRNA. ( b ) qRT–PCR for the Notch pathway targets Hes1 and Hey1 in WT and Nuc1 astrocytes after treatment with scrambled or Jagged1 siRNA. Knockdown of Jagged1 expression (* P =0.013 in WT and * P =0.017 in Nuc1) is reflected by decreased expression of Hes1 (* P =0.022 in WT and * P =0.015 in Nuc1) and Hey1 (right panel: values relative to scrambled siRNA in left panel). ( c ) 12XCSL-luciferase reporter activity in cocultures of Notch1-expressing astrocytes carrying 12XCSL-luciferase reporter construct (ΔEGF) or pRL-cmv control (EGF) construct, with astrocytes overexpressing the Jagged1 ligand. Graph shows luciferase activity (arithmetic mean) from triplicates of each coculture. Robust luciferase activity was seen in WT astrocytes (* P =0.011), compared with Nuc1 astrocytes. This increase is compromised in astrocytes expressing the Jagged1 ΔEGF Notch-binding-deficient plasmid. ( d ) 12XCSL-luciferase reporter activity in cocultures of Jagged1 knockdown astrocytes expressing 12XCSL-luciferase reporter construct or pRL-cmv control constructs with astrocytes overexpressing Jagged1. A marked induction of Notch signalling was observed in both WT (* P =0.019) and Nuc1 astrocytes transfected with Jagged1 siRNA (* P =0.027) and cocultured with astrocytes overexpressing Jagged1 compared with scrambled siRNA-treated cells (left panel). Astrocytes transfected with empty vector were also cocultured with Jagged1 overexpressing cells, showing a modest induction of the Notch pathway in WT and none in Nuc1 homozygous astrocytes. In all panels, graphs show mean values and error bars represent s.d. from a triplicate experiment representative of at least three independent experiments. Statistical analysis was performed by a two-tailed Student’s t -test: * P <0.05. Full size image To study the Jagged1-mediated activation of Notch signalling, we used a coculture system where cells expressing full-length Notch1 receptor and the 12XCSL-luciferase Notch reporter and pRL-CMV renilla plasmids were interfaced with cells expressing full-length Jagged1. We observed robust 12XCSL-luciferase activation in WT cells, whereas Nuc1 cells showed much weaker activation of the Notch pathway ( Fig. 3c ). As control, a vector expressing a mutant Jagged1 protein that fails to bind to the Notch receptor (Jagged1ΔEGF) was used. This resulted in an abrogation of Notch signalling, suggesting that the trans -interactions with Jagged1-expressing cells were inhibited. As optic nerve astrocytes express both Notch1 and Jagged1, we next asked whether the Notch receptor is cis -inhibited by ligand expressed in the same cell and trans -activated by ligand expressed on neighbouring cells. In most cancer cells, Notch receptor and ligand are expressed by the same cell, with the ligand inhibiting the receptor, thereby facilitating the receptor trans -interaction with ligand expressed by neighbouring cells [29] . We studied the trans -interactions by silencing Jagged1 expression using siRNA and transfecting the same cells with the 12XCSL-luciferase Notch reporter plasmid and pRL-CMV Renilla plasmid. Figure 3d shows significant induction of Notch signalling in both WT and Nuc1 astrocytes, suggesting a cis -inhibition of the receptor by Jagged1 in the same cell and trans -activation by Jagged1 on neighbouring cells. Cells transfected with non-targeting siRNA were also cocultured with Jagged1 overexpressing cells, showing only a modest induction of the Notch pathway in WT, and none in Nuc1 astrocytes ( Fig. 3d ). Defective S3 cleavage decreases NICD in Nuc1 astrocytes Our data show that NICD is decreased in Nuc1 cells despite the higher levels of Notch1 receptor. As this could result from defective proteolytic cleavage of Notch, we analysed the two cleavage steps required for Notch activation. The S2 and S3 cleavages are mediated by ADAM metalloprotease and γ-secretase, respectively [5] . In cells treated with a hydroxamate ADAM inhibitor, BB-94, the mRNA expression of Notch targets Hes1 and Hey1 was inhibited in both WT and Nuc1 cells ( Fig. 4a ). To confirm cleavage of the Notch receptor, we used a myc-tagged, constitutively active, membrane-bound derivative of Notch1 (NδE). Cleavage of NδE at V1744 by γ-secretase generates a product corresponding to NICD. This construct was visualized by immunoblotting with anti-Myc antibody. In both WT and Nuc1 optic nerve astrocytes expressing NδE, an ~85-kDa protein representing uncleaved NδE and a 75-kDa band corresponding to NICD were detected. 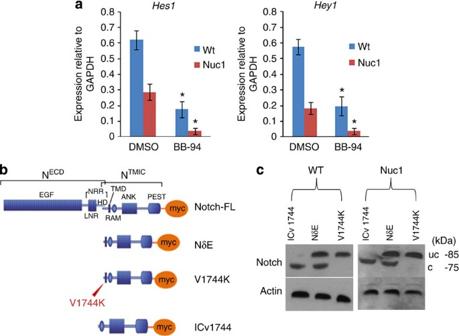Figure 4: Proteolytic cleavage of Notch in WT and Nuc1 astrocytes. (a) WT and Nuc1 astrocytes were treated with the metalloproteinase inhibitor BB-94 and expression of the Notch target genes,Hes1andHey1, determined by qRT–PCR. Expression of these genes was decreased to similar extent in WT(Hes1*P=0.031 andHey1*P=0.022) and Nuc1 astrocytes (Hes1*P=0.027 andHey1*P=0.027), (BB-94 relative to dimethylsulphoxide (DMSO)). (b) Depiction of Notch plasmids (modified from Ilaganet al.60) used to define Notch cleavage. At top is shown the myc-tagged full-length Notch (Notch-FL). NδE denotes the constitutively active, membrane-bound derivative of Notch1 that was produced by deletion of the EGF repeats. V1744K is the NδE-derived construct with a mutation at the Notch cleavage site (V1774K), preventing the cleavage and release of the NICD. ICv1744 is also an NδE-derived construct that is truncated at the cleavage site thereby generating only cleaved Notch. (c) Nuc1 astrocytes were transfected with a Myc epitope-tagged constitutively active Notch plasmid, NδE. Cells were also transfected with NδE (V1744K) with a mutation at the cleavage site generating a non-cleavable form of Notch, and with ICv1744, a truncated Notch plasmid that expresses only the cleaved form of Notch. Western analysis was performed with monoclonal anti-Myc antibody. The uncleaved (uc) and cleaved (c) forms of Notch were identified as bands corresponding to ~85 kDa and ~75 kDa, respectively. Both the uc and c bands were identified in WT and Nuc1 astrocytes transfected with NδE. NδE (V1744K) and ICv1744 plasmids served as controls for the uc and c forms, respectively. In all panels, graphs show mean values and error bars represent s.d. from a triplicate experiment representative of at least three independent experiments. Statistical analysis was performed by a two-tailed Student’st-test: *P<0.05. Figure 4: Proteolytic cleavage of Notch in WT and Nuc1 astrocytes. ( a ) WT and Nuc1 astrocytes were treated with the metalloproteinase inhibitor BB-94 and expression of the Notch target genes, Hes1 and Hey1 , determined by qRT–PCR. Expression of these genes was decreased to similar extent in WT (Hes1 * P =0.031 and Hey1 * P =0.022) and Nuc1 astrocytes ( Hes1 * P =0.027 and Hey1 * P =0.027), (BB-94 relative to dimethylsulphoxide (DMSO)). ( b ) Depiction of Notch plasmids (modified from Ilagan et al. [60] ) used to define Notch cleavage. At top is shown the myc-tagged full-length Notch (Notch-FL). NδE denotes the constitutively active, membrane-bound derivative of Notch1 that was produced by deletion of the EGF repeats. V1744K is the NδE-derived construct with a mutation at the Notch cleavage site (V1774K), preventing the cleavage and release of the NICD. ICv1744 is also an NδE-derived construct that is truncated at the cleavage site thereby generating only cleaved Notch. ( c ) Nuc1 astrocytes were transfected with a Myc epitope-tagged constitutively active Notch plasmid, NδE. Cells were also transfected with NδE (V1744K) with a mutation at the cleavage site generating a non-cleavable form of Notch, and with ICv1744, a truncated Notch plasmid that expresses only the cleaved form of Notch. Western analysis was performed with monoclonal anti-Myc antibody. The uncleaved (uc) and cleaved (c) forms of Notch were identified as bands corresponding to ~85 kDa and ~75 kDa, respectively. Both the uc and c bands were identified in WT and Nuc1 astrocytes transfected with NδE. NδE (V1744K) and ICv1744 plasmids served as controls for the uc and c forms, respectively. In all panels, graphs show mean values and error bars represent s.d. from a triplicate experiment representative of at least three independent experiments. Statistical analysis was performed by a two-tailed Student’s t -test: * P <0.05. Full size image To confirm the identity of these fragments, WT and Nuc1 astrocytes were first transfected with a NδE construct mutated at residue 1,744 (V1744K) to prevent cleavage and generate a band comigrating with the higher-molecular-mass NδE band. Further, astrocytes transfected with an NδE-derived construct truncated at the cleavage site (ICv1744), produced a fragment comigrating with NICD ( Fig. 4b ). As both the cleaved and uncleaved forms were generated in Nuc1 astrocytes expressing NδE, the cleavage sites of Notch1 are functional in the mutant astrocytes. NICD translocation occurs normally in Nuc1 astrocytes We next investigated whether nuclear translocation of NICD is inhibited in Nuc1 astrocytes. For this, we overexpressed NICD in WT and Nuc1 astrocytes using a constitutively active Notch1 construct in a pCDNA3.1 plasmid. Overexpression was confirmed by western analysis ( Fig. 5a ). Increased staining for NICD was seen in both WT and Nuc1 astrocytes compared with astrocytes transfected with vector alone ( Fig. 5b ). qRT–PCR showed that overexpression of NICD by Nuc1 astrocytes strongly rescued expression of Notch target genes ( Fig. 5c ). The expression of Hey1 and Hes1 was also measured in WT and Nuc1 cells transfected with Notch-FL and Notch extracellular truncation plasmids. In contrast to overexpression of NICD, neither of these constructs rescued Hey1 or Hes1 expression in Nuc1 astrocytes ( Fig. 5d ). 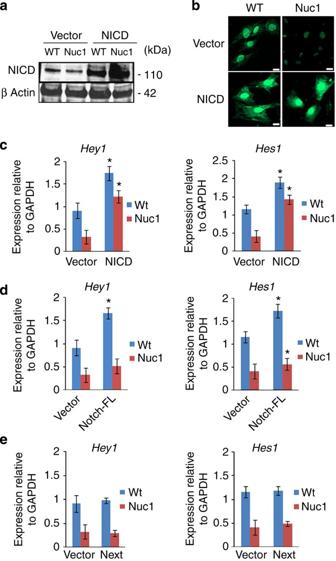Figure 5: Nuclear translocation of active Notch. (a) WT and Nuc1 astrocytes transfected with the NICD overexpression construct or vector control were immunoblotted with Notch anti-V1744 antibody to detect NICD. Elevated levels of NICD were seen in both WT and Nuc1 astrocytes transfected with the NICD overexpression construct compared with vector-transfected astrocytes. (b) Immunostaining of NICD-transfected and vector-transfected WT and Nuc1 astrocytes with Notch anti-V1744 antibody detected increased nuclear staining of NICD in NICD-transfected astrocytes compared with vector-transfected astrocytes. Scale bar, 20 μm. (c) qRT–PCR to detect the expression levels ofHey1andHes1in WT and Nuc1 astrocytes transfected with NICD or vector only. NICD-transfected Nuc1 astrocytes showed a rescue in the expression of bothHey1andHes1(*P=0.012; *P=0.017. respectively). (d,e) qRT-PCR to detect the expression levels ofHey1andHes1in cells transfected with Notch full length (Notch-FL) showed increased expression ofHey1(*P=0.026; *P=0.017) andHes1(*P=0.031; *P=0.017) in WT astrocytes, but not in Nuc1 astrocytes. No changes in the expression ofHey1andHes1were observed in both the cell types transfected with Notch extracellular truncation domain (NEXT) plasmids. In all panels, graphs show mean values and error bars represent s.d. from a triplicate experiment representative of at least three independent experiments. Statistical analysis was performed by a two-tailed Student’st-test: *P<0.05. Figure 5: Nuclear translocation of active Notch. ( a ) WT and Nuc1 astrocytes transfected with the NICD overexpression construct or vector control were immunoblotted with Notch anti-V1744 antibody to detect NICD. Elevated levels of NICD were seen in both WT and Nuc1 astrocytes transfected with the NICD overexpression construct compared with vector-transfected astrocytes. ( b ) Immunostaining of NICD-transfected and vector-transfected WT and Nuc1 astrocytes with Notch anti-V1744 antibody detected increased nuclear staining of NICD in NICD-transfected astrocytes compared with vector-transfected astrocytes. Scale bar, 20 μm. ( c ) qRT–PCR to detect the expression levels of Hey1 and Hes1 in WT and Nuc1 astrocytes transfected with NICD or vector only. NICD-transfected Nuc1 astrocytes showed a rescue in the expression of both Hey1 and Hes1 (* P =0.012; * P =0.017. respectively). ( d , e ) qRT-PCR to detect the expression levels of Hey1 and Hes1 in cells transfected with Notch full length (Notch-FL) showed increased expression of Hey1 (* P =0.026; * P =0.017) and Hes1 (* P =0.031; * P =0.017) in WT astrocytes, but not in Nuc1 astrocytes. No changes in the expression of Hey1 and Hes1 were observed in both the cell types transfected with Notch extracellular truncation domain (NEXT) plasmids. In all panels, graphs show mean values and error bars represent s.d. from a triplicate experiment representative of at least three independent experiments. Statistical analysis was performed by a two-tailed Student’s t -test: * P <0.05. Full size image βA3/A1-crystallin regulates γ-secretase activity γ-Secretase is enzymatically more active in the low pH environment of the endolysosomal compartments [9] , [30] . In the case of amyloid precursor protein, a well-characterized γ-secretase substrate, cleavage to produce β-amyloid occurs in the endolysosomal compartments [31] . To determine whether the activity and subcellular distribution of γ-secretase is aberrant in Nuc1 astrocytes, postnuclear supernatants (PNSs) from WT and Nuc1 astrocytes were layered on iodixanol gradients and subjected to ultracentrifugation. The composition of the fractions was determined by immunoblotting with specific markers. Lysosome-associated membrane protein1 (LAMP1)-positive lysosomes were strongest in fractions 3, 4 and 5; Rab5-positive endosomes in fractions 6, 7 and 8; and Golgi in fractions 9 and 10 ( Fig. 6a ). The activity of γ-secretase was measured by performing ELISA to quantify production of β-amyloid 40. In WT astrocytes, γ-secretase activity ( Fig. 6b ) was present in fractions 3, 4 and 5 corresponding to the lysosomes; fractions 6, 7 and 8 corresponding to the Rab5-positive endosomes. We also detected modest activity in the Golgi. Nuc1 astrocytes showed significantly decreased γ-secretase activity in the endolysosomal compartments, whereas activity in the Golgi was relatively unchanged ( Fig. 6c ). Overexpression of βA3/A1-crystallin in Nuc1 astrocytes restored normal γ-secretase activity ( Fig. 6d ). To confirm that βA3/A1-crystallin modulates γ-secretase activity in astrocytes, we performed Cryba1 siRNA-silencing studies to downregulate βA3/A1-crystallin in WT rat astrocytes in culture using specific ON-TARGET plus SMART pool siRNA (Dharmacon, CO). Scrambled siRNA was used as control. Knockdown of βA3/A1-crystallin in WT astrocytes decreases γ-secretase activity, but the decrease is not as robust as in Nuc1 homozygous astrocytes, the activity could be rescued to normal levels by subsequent overexpression of βA3/A1-crystallin ( Supplementary Fig. S1 ). As proof of principle that βA3/A1-crystallin can modulate γ-secretase activity in astrocytes, we used Nuc1 heterozygote astrocytes in culture and downregulated βA3/A1-crystallin with siRNA as above. The concentration of siRNA required to downregulate Cryba1 in Nuc1 heterozygotes was significantly lower than that needed with WT astrocytes. Heterozygote astrocytes in which Cryba1 was downregulated showed loss of γ-secretase activity to levels similar to that in Nuc1 homozygous astrocytes. Activity was rescued by overexpression of βA3/A1-crystallin in the same cells ( Fig. 6e ). In addition, Cryba1 -floxed mice were generated ( Supplementary Fig. S2 ); downregulation of βA3/A1-crystallin in astrocytes cultured from these mice, using an adenoviral vector expressing Cre-recombinase, also decreased γ-secretase activity, however, this activity was rescued by subsequent overexpression of βA3/A1-crystallin ( Fig. 6f ). γ-Secretase activity was also decreased in endolysosomes of both WT and Nuc1 astrocytes pretreated with chloroquine, an inhibitor of lysosomal acidification ( Supplementary Fig. S3 ). The decrease in activity was more significant in WT astrocytes than in Nuc1. γ-Secretase activity was not affected in Golgi, a non-acidic compartment. Previous studies, and our results, indicate a stringent pH requirement for γ-secretase activity [12] , [31] , [32] . Although low levels of γ-secretase activity are detectable in Nuc1 astrocytes, that activity may be insufficient for optimal Notch signalling. Previous studies in other systems have shown that treatment with DAPT resulted in a marked decrease in the generation of NICD, as monitored by expression of Hey1 and Hes1 (refs 5 , 33 ). qRT–PCR analysis revealed that DAPT treatment reduced Hes1 and Hey1 similarly in WT and Nuc1 cells ( Supplementary Fig. S4 ). 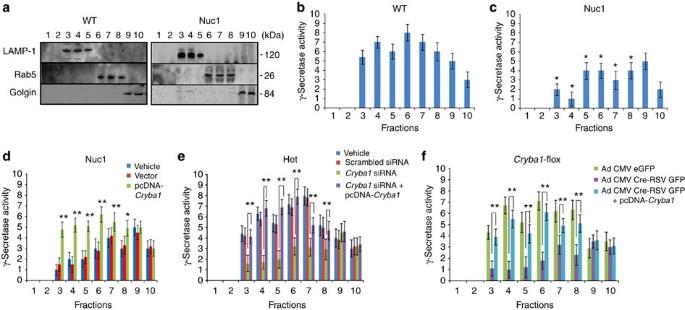Figure 6: Assessment of γ-secretase activity in WT and in astrocytes lacking βA3/A1-crystallin. (a) Post-mitochondrial supernatants from WT and Nuc1 astrocytes were layered on 2.5–30% iodixanol gradients and subjected to ultracentrifugation. Western blots identified LAMP1-positive lysosomes in fractions 3, 4 and 5; Rab5-positive endosomes in fractions 6, 7 and 8; and Golgi in fractions 9 and 10. (b) ELISA was performed to quantify β-amyloid (Aβ40) production after incubating above fractions overnight at 37 °C, with or without L-685,458 (γ-secretase inhibitor). In WT astrocytes, γ-secretase activity, as measured by Aβ40 level, was detected in fractions 3, 4 and 5 (lysosomes), and in fractions 6, 7 and 8 (late and early endosomes). γ-Secretase activity was detected at lower level in the Golgi (fractions 9 and 10). (c) In Nuc1 astrocytes, γ-secretase activity was significantly decreased in the endolysosomal compartments (~50% reduction), whereas the activity in Golgi was unchanged. (d) Overexpression of βA3/A1-crystallin in astrocytes cultured from Nuc1 rats rescued γ-secretase activity in endolysosomal compartments, while empty vector had no effect (relative to vehicle). (e) Deletion ofCryba1from Nuc1 heterozygote astrocytes using aCryba1ON-TARGET-plus SMART pool siRNA reduced γ-secretase activity in endolysosomal compartments substantially to levels comparable to that of Nuc1 homozygote astrocytes. There was no effect on activity in Golgi. Overexpression of βA3/A1-crystallin in the same astrocytes, as ine, rescued activity to control levels in the endolysosomal fractions. Scrambled siRNA had no effect (relative to vehicle). (f) Astrocytes fromCryba1-floxed mice were infected with recombinant adenovirus (Ad) constructs (Ad CMV Cre-RSV GFP or Ad CMV-eGFP) followed by βA3/A1-crystallin overexpression.Cryba1-knockout (Ad CMV Cre-RSV GFP) mouse astrocytes show markedly reduced γ-secretase activity in the endolysosomal compartments, with no effect on Golgi. Subsequent overexpression of βA3/A1-crystallin rescued activity to near-normal levels in endolysosomal fractions (relative toCryba1flox-Ad CMV-eGFP). In all panels, graphs show mean values and error bars represent s.d. from a triplicate experiment representative of at least three independent experiments. Statistical analysis was performed by a two-tailed Student’st-test: *P<0.05; **P<0.01. Figure 6: Assessment of γ-secretase activity in WT and in astrocytes lacking βA3/A1-crystallin. ( a ) Post-mitochondrial supernatants from WT and Nuc1 astrocytes were layered on 2.5–30% iodixanol gradients and subjected to ultracentrifugation. Western blots identified LAMP1-positive lysosomes in fractions 3, 4 and 5; Rab5-positive endosomes in fractions 6, 7 and 8; and Golgi in fractions 9 and 10. ( b ) ELISA was performed to quantify β-amyloid (Aβ40) production after incubating above fractions overnight at 37 °C, with or without L-685,458 (γ-secretase inhibitor). In WT astrocytes, γ-secretase activity, as measured by Aβ40 level, was detected in fractions 3, 4 and 5 (lysosomes), and in fractions 6, 7 and 8 (late and early endosomes). γ-Secretase activity was detected at lower level in the Golgi (fractions 9 and 10). ( c ) In Nuc1 astrocytes, γ-secretase activity was significantly decreased in the endolysosomal compartments (~50% reduction), whereas the activity in Golgi was unchanged. ( d ) Overexpression of βA3/A1-crystallin in astrocytes cultured from Nuc1 rats rescued γ-secretase activity in endolysosomal compartments, while empty vector had no effect (relative to vehicle). ( e ) Deletion of Cryba1 from Nuc1 heterozygote astrocytes using a Cryba1 ON-TARGET-plus SMART pool siRNA reduced γ-secretase activity in endolysosomal compartments substantially to levels comparable to that of Nuc1 homozygote astrocytes. There was no effect on activity in Golgi. Overexpression of βA3/A1-crystallin in the same astrocytes, as in e , rescued activity to control levels in the endolysosomal fractions. Scrambled siRNA had no effect (relative to vehicle). ( f ) Astrocytes from Cryba1 -floxed mice were infected with recombinant adenovirus (Ad) constructs (Ad CMV Cre-RSV GFP or Ad CMV-eGFP) followed by βA3/A1-crystallin overexpression. Cryba1 -knockout (Ad CMV Cre-RSV GFP) mouse astrocytes show markedly reduced γ-secretase activity in the endolysosomal compartments, with no effect on Golgi. Subsequent overexpression of βA3/A1-crystallin rescued activity to near-normal levels in endolysosomal fractions (relative to Cryba1 flox-Ad CMV-eGFP). In all panels, graphs show mean values and error bars represent s.d. from a triplicate experiment representative of at least three independent experiments. Statistical analysis was performed by a two-tailed Student’s t -test: * P <0.05; ** P <0.01. Full size image βA3/A1-crystallin affects V-ATPase activity As γ-secretase activity is compromised in astrocytes lacking functional βA3/A1-crystallin, we suspected that endolysosomal acidification might be dysregulated. To obtain direct evidence that this may be the case, we compared V-ATPase activity in astrocytes lacking βA3/A1-crystallin with WT. Isolated lysosomes were incubated in acridine orange and accumulation of protonated acridine in the lysosomes measured by the resultant fluorescence. In the presence of exogenous ATP, H + uptake was significantly increased in the lysosomes of WT astrocytes. Under the same conditions, the acridine orange fluorescence in Nuc1 astrocytes was significantly lower ( Fig. 7a ). V-ATPase activity in Nuc1 homozygote astrocytes was rescued by βA3/A1-crystallin overexpression ( Fig. 7b ). We further demonstrate reduced V-ATPase activity in βA3/A1-crystallin-downregulated Nuc1 heterozygote astrocytes ( Fig. 7c ), and in astrocytes isolated from Cryba1 -floxed mice, after βA3/A1-crystallin deletion ( Fig. 7d ). Moreover, the V-ATPase activity could be rescued by subsequent overexpression of βA3/A1-crystallin ( Fig. 7c ). Endolysosomal pH was measured by monitoring fluorescence changes in astrocytes loaded with fluorescein isothiocyanate (FITC)-dextran. In WT the average endolysosomal pH was 4.5, increasing to 5.7 in Nuc1 astrocytes ( Fig. 7e ). This increase in pH was reversed by overexpression of βA3/A1-crystallin in the same cells ( Fig. 7f ). Similarly, loss of βA3/A1-crystallin in Nuc1 heterozygote and Cryba1 -floxed astrocytes induced alkalinization by ~1 pH unit and was rescued to near-normal levels by subsequent overexpression of βA3/A1-crystallin in the same astrocytes ( Fig. 7g ), suggesting a direct role of βA3/A1-crystallin in regulating acidification of astrocytes. 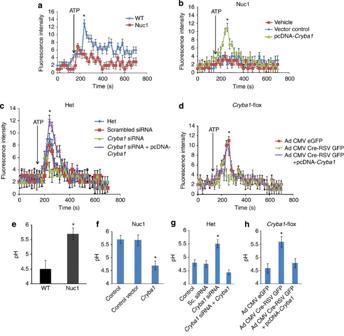Figure 7: Impaired V-ATPase activity in astrocytes lacking functional βA3/A1-crystallin. (a) V-ATPase activity was measured by acridine orange fluorescence in WT and Nuc1 astrocytes after intravesicular H+uptake was initiated by the addition of Mg-ATP. Increase in acridine orange fluorescence upon addition of ATP was significantly greater in WT astrocytes compared with Nuc1 astrocytes (*P=0.017). During the measurement of lysosomal pH, bafilomycin a1 was added to the ATP-treated lysosomes for control purposes. (b) In Nuc1 astrocytes, overexpression of βA3/A1-crystallin rescued activity to >80% of normal level (*P=0.020). Empty vector had no effect. (c) V-ATPase activity in heterozygote astrocytes was significantly reduced byCryba1siRNA knockdown (*P=0.033), but was rescued to normal levels when βA3/A1-crystallin was subsequently overexpressed in the same astrocytes (*P=0.024). (d) In astrocytes from mice with floxedCryba1, deletion ofCryba1by Cre-recombinase decreased V-ATPase activity relative to control astrocytes (*P=0.018). The V-ATPase activity was rescued to normal levels by subsequent overexpression of βA3/A1-crystallin inCryba1-knockout mouse astrocytes (*P=0.027). (e) Measurement of endolysosomal pH in WT and Nuc1 astrocytes was performed using a fluid-phase fluorescent probe, FITC-dextran. Three hours after incubation of WT and Nuc1 astrocytes with FITC-dextran, the fluorescence emission was measured at 520 nm with excitation at 450 nm and 495 nm. The fluorescence excitation ratio at 495 nm and 450 nm (I495nm/I450nm) was calculated, and endolysosomal pH in WT and Nuc1 astrocytes was measured to be ~4.5 and 5.7, respectively (*P=0.031). (f) The elevated pH in Nuc1 homozygous astrocytes was restored to near-normal acidic range by overexpression of βA3/A1-crystallin (*P=0.026). Empty vector had no effect. (g) Further knockdown of βA3/A1-crystallin in Nuc1 heterozygote astrocytes byCryba1siRNA elevated the endolysosomal pH to near Nuc1 homozygous levels (*P=0.036). Subsequent overexpression of βA3/A1-crystallin decreased pH to the level characteristic of WT astrocytes (*P=0.021). Scrambled siRNA had no effect. (h) pH was elevated to near Nuc1 homozygote level inCryba1-knockout mouse astrocytes (*P=0.029) and was rescued to near-normal levels by subsequent overexpression of βA3/A1-crystallin to same cells (*P=0.024). In all panels, graphs show mean values and error bars represent s.d. from a triplicate experiment representative of at least three independent experiments. Statistical analysis was performed by a two-tailed Student’st-test: *P<0.05. Figure 7: Impaired V-ATPase activity in astrocytes lacking functional βA3/A1-crystallin. ( a ) V-ATPase activity was measured by acridine orange fluorescence in WT and Nuc1 astrocytes after intravesicular H + uptake was initiated by the addition of Mg-ATP. Increase in acridine orange fluorescence upon addition of ATP was significantly greater in WT astrocytes compared with Nuc1 astrocytes (* P =0.017). During the measurement of lysosomal pH, bafilomycin a1 was added to the ATP-treated lysosomes for control purposes. ( b ) In Nuc1 astrocytes, overexpression of βA3/A1-crystallin rescued activity to >80% of normal level (* P =0.020). Empty vector had no effect. ( c ) V-ATPase activity in heterozygote astrocytes was significantly reduced by Cryba1 siRNA knockdown (* P =0.033), but was rescued to normal levels when βA3/A1-crystallin was subsequently overexpressed in the same astrocytes (* P =0.024). ( d ) In astrocytes from mice with floxed Cryba1 , deletion of Cryba1 by Cre-recombinase decreased V-ATPase activity relative to control astrocytes (* P =0.018). The V-ATPase activity was rescued to normal levels by subsequent overexpression of βA3/A1-crystallin in Cryba1 -knockout mouse astrocytes (* P =0.027). ( e ) Measurement of endolysosomal pH in WT and Nuc1 astrocytes was performed using a fluid-phase fluorescent probe, FITC-dextran. Three hours after incubation of WT and Nuc1 astrocytes with FITC-dextran, the fluorescence emission was measured at 520 nm with excitation at 450 nm and 495 nm. The fluorescence excitation ratio at 495 nm and 450 nm ( I 495nm / I 450nm ) was calculated, and endolysosomal pH in WT and Nuc1 astrocytes was measured to be ~4.5 and 5.7, respectively (* P =0.031). ( f ) The elevated pH in Nuc1 homozygous astrocytes was restored to near-normal acidic range by overexpression of βA3/A1-crystallin (* P =0.026). Empty vector had no effect. ( g ) Further knockdown of βA3/A1-crystallin in Nuc1 heterozygote astrocytes by Cryba1 siRNA elevated the endolysosomal pH to near Nuc1 homozygous levels (* P =0.036). Subsequent overexpression of βA3/A1-crystallin decreased pH to the level characteristic of WT astrocytes (* P =0.021). Scrambled siRNA had no effect. ( h ) pH was elevated to near Nuc1 homozygote level in Cryba1 -knockout mouse astrocytes (* P =0.029) and was rescued to near-normal levels by subsequent overexpression of βA3/A1-crystallin to same cells (* P =0.024). In all panels, graphs show mean values and error bars represent s.d. from a triplicate experiment representative of at least three independent experiments. Statistical analysis was performed by a two-tailed Student’s t -test: * P <0.05. Full size image Degradation of Notch receptor is impaired in Nuc1 astrocytes As defective acidification of endolysosomal compartments could also lead to impaired degradation of Notch, we compared the clearance of the Notch receptor in WT and Nuc1 astrocytes after transfection with the Myc-tagged full-length Notch1 receptor. To activate the Notch pathway, these cells were cocultured with cells overexpressing Jagged1. After 1 h, the myc-tagged Notch1 underwent significant clearance from the cytosol in WT astrocytes. In Nuc1 astrocytes, however, Notch1 strongly persisted. After 3 h, most of the tagged receptor was degraded in WT, but much remained in the perinuclear region of Nuc1 astrocytes ( Fig. 8a ). 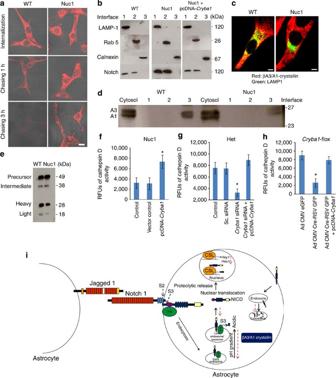Figure 8: Intracellular processing and degradation of Notch receptor. (a) WT and Nuc1 astrocytes transfected with myc-tagged full-length Notch1 receptor were monitored for receptor clearance when cocultured with astrocytes overexpressing Jagged1. Top panels show myc labelling (red) after transfection. Labelling decreased quickly in WT astrocytes, with little remaining after 3 h. Degradation was minimal in the Nuc1 astrocytes. Scale bar, 20 μm. (b) Subcellular fractionation showed Notch1 present in LAMP1-positive late endosomes/lysosomes (interface 1) and Rab5-positive early endosomes (interface 2) in both WT and Nuc1 astrocytes, but more strongly so in Nuc1. Overexpression of βA3/A1-crystallin in Nuc1 astrocytes (right panel) stimulated Notch1 degradation, decreasing Notch1 to the range present in WT astrocytes. Notch1 was not present in endoplasmic reticulum (calnexin-positive lane). (c) Immunostaining of WT and Nuc1 astrocytes for βA3/A1-crystallin (red), revealed abundant staining in the cytosol in both cell types. Co-localization (yellow) with LAMP1-positive lysosomes (green) was perinuclear in WT; little co-localization was seen in Nuc1 and lysosome distribution was abnormal. Scale bar, 20 μm. (d) Subcellular fractionation revealed both βA3- and βA1-crystallins in the cytosol of WT and Nuc1 astrocytes. They were more strongly associated with lysosomes (Interface 1) in WT astrocytes. (e) Western analysis demonstrated substantially reduced levels of Cathepsin D heavy (~50%) and light (~60%) chains in Nuc1 homozygote astrocytes relative to WT, consistent with decreased active enzyme in the mutant astrocytes. Quantification as described in Methods. (f) Overexpression of βA3/A1-crystallin in Nuc1 astrocytes increased activity from 30 to 75% of WT level (*P=0.037). (g) Cathepsin D activity in Nuc1 heterozygote astrocytes was decreased 80% byCryba1siRNA knockdown of βA3/A1-crystallin (**P=0.011); subsequent overexpression of βA3/A1-crystallin rescued activity to control values (**P=0.009). (h) In astrocytes fromCryba1-floxed mice, deletion by Cre-recombinase reduced Cathepsin D activity (~60%) (*P=0.031); subsequent overexpression of βA3/A1-crystallin rescued the activity (*P=0.018). (i) Schematic model of Notch signalling and βA3/A1-crystallin. Steps affected by loss of βA3/A1-crystallin shown by red dotted arrows. Impaired endolysosomal acidification inhibits Notch receptor processing and degradation, decreases NICD, ultimately reducing transcription of Notch target genes. In all panels, graphs show mean values and error bars represent s.d. from a triplicate experiment representative of at least three independent experiments. Statistical analysis was performed by a two-tailed Student’st-test: **P<0.01; *P<0.05. Figure 8: Intracellular processing and degradation of Notch receptor. ( a ) WT and Nuc1 astrocytes transfected with myc-tagged full-length Notch1 receptor were monitored for receptor clearance when cocultured with astrocytes overexpressing Jagged1. Top panels show myc labelling (red) after transfection. Labelling decreased quickly in WT astrocytes, with little remaining after 3 h. Degradation was minimal in the Nuc1 astrocytes. Scale bar, 20 μm. ( b ) Subcellular fractionation showed Notch1 present in LAMP1-positive late endosomes/lysosomes (interface 1) and Rab5-positive early endosomes (interface 2) in both WT and Nuc1 astrocytes, but more strongly so in Nuc1. Overexpression of βA3/A1-crystallin in Nuc1 astrocytes (right panel) stimulated Notch1 degradation, decreasing Notch1 to the range present in WT astrocytes. Notch1 was not present in endoplasmic reticulum (calnexin-positive lane). ( c ) Immunostaining of WT and Nuc1 astrocytes for βA3/A1-crystallin (red), revealed abundant staining in the cytosol in both cell types. Co-localization (yellow) with LAMP1-positive lysosomes (green) was perinuclear in WT; little co-localization was seen in Nuc1 and lysosome distribution was abnormal. Scale bar, 20 μm. ( d ) Subcellular fractionation revealed both βA3- and βA1-crystallins in the cytosol of WT and Nuc1 astrocytes. They were more strongly associated with lysosomes (Interface 1) in WT astrocytes. ( e ) Western analysis demonstrated substantially reduced levels of Cathepsin D heavy (~50%) and light (~60%) chains in Nuc1 homozygote astrocytes relative to WT, consistent with decreased active enzyme in the mutant astrocytes. Quantification as described in Methods. ( f ) Overexpression of βA3/A1-crystallin in Nuc1 astrocytes increased activity from 30 to 75% of WT level (* P =0.037). ( g ) Cathepsin D activity in Nuc1 heterozygote astrocytes was decreased 80% by Cryba1 siRNA knockdown of βA3/A1-crystallin (** P =0.011); subsequent overexpression of βA3/A1-crystallin rescued activity to control values (** P =0.009). ( h ) In astrocytes from Cryba1 -floxed mice, deletion by Cre-recombinase reduced Cathepsin D activity (~60%) (* P =0.031); subsequent overexpression of βA3/A1-crystallin rescued the activity (* P =0.018). ( i ) Schematic model of Notch signalling and βA3/A1-crystallin. Steps affected by loss of βA3/A1-crystallin shown by red dotted arrows. Impaired endolysosomal acidification inhibits Notch receptor processing and degradation, decreases NICD, ultimately reducing transcription of Notch target genes. In all panels, graphs show mean values and error bars represent s.d. from a triplicate experiment representative of at least three independent experiments. Statistical analysis was performed by a two-tailed Student’s t -test: ** P <0.01; * P <0.05. Full size image As degradation of Notch1 appeared dysfunctional in Nuc1 astrocytes, we performed subcellular fractionation using sucrose density gradients. Notch1 was found at interfaces 1 and 2, containing LAMP1-positive lysosomes and Rab5-positive early endosomes, respectively ( Fig. 8b ). The Nuc1 homozygote astrocytes showed greater accumulation of Notch1 in these compartments than did WT astrocytes, suggesting that Nuc1 cells have a compromised ability to degrade and process the Notch receptor. Moreover, overexpression of βA3/A1-crystallin in Nuc1 homozygote astrocytes restored normal lysosomal-mediated degradation of Notch ( Fig. 8b ). As Nuc1 results from a mutation in βA3/A1-crystallin, we also determined the subcellular localization of βA3/A1-crystallin in astrocytes. Immunostaining revealed that while βA3/A1-crystallin was predominantly cytosolic in both WT and Nuc1 astrocytes, it also co-localized with LAMP1-positive lysosomes in WT astrocytes and, to a lesser extent, in Nuc1 astrocytes ( Fig. 8c ). Western analysis of the sucrose gradient fractions confirmed these results ( Fig. 8d ). Our results demonstrate that βA3/A1-crystallin is required for normal lysosomal acidification. To determine whether βA3/A1-crystallin also modulates the activity of lysosomal enzymes, we assayed the activity of Cathepsin D, a lysosomal hydrolase requiring low pH for optimal activity. The intermediate chain of Cathepsin D is processed into the active heavy and light chains once the protein encounters the acidic lysosomal environment. Changes in this processing reflect altered function of lysosomal hydrolases. Levels of both the heavy and light chains were decreased in Nuc1 homozygote astrocytes ( Fig. 8e ) and Cathepsin D activity was rescued by overexpression of βA3/A1-crystallin ( Fig. 8f ). Our data also indicate that in Nuc1 heterozygotes and in Cryba1 -floxed astrocytes, Cathepsin D activity was markedly reduced, while subsequent overexpression of βA3/A1-crystallin rescued activity ( Fig. 8g ). Functional effects of Cryba1 knockout from Cryba1 -floxed mouse astrocytes are demonstrated above ( Figs 6 , 7 , 8 ). To prove that Notch signalling is affected, we measured Hes1 and Hey1 expression, finding it decreased in the Cre-infected astrocytes and rescued by subsequent overexpression of βA3/A1-crystallin ( Supplementary Fig. S5 ). To determine whether compromise of the ubiquitin-proteosome system in Nuc1 astrocytes might affect Notch degradation, we measured the intracellular levels of the receptor in the presence of specific inhibitors of the ubiquitin proteosomal pathway, clasto-lactacystin β-lactone and MG132 (ref. 34 ). Treatment with neither inhibitor resulted in a significant accumulation of Notch1 receptor in WT or Nuc1 homozygote astrocytes ( Supplementary Fig. S6 ). Thus, our results suggest that in astrocytes, endogenous Notch receptor is posttranslationally regulated predominantly by the lysosomal-mediated degradative pathway. Impaired Notch signalling reduces GFAP promoter activity Notch signalling has been implicated in the demethylation and activation of the GFAP promoter [35] . As GFAP is an important factor in astroglial differentiation [35] and as the astrocyte template in the Nuc1 homozygote retina is abnormal, we wondered whether Nuc1 astrocytes differentiated normally. To determine whether Notch is involved in the transcriptional regulation of GFAP in optic nerve astrocytes, we assayed GFAP promoter activity using a GFAP promoter–reporter construct containing the rat GFAP promoter upstream of the firefly luciferase cDNA and the Renilla luciferase reporter under the control of CMV promoter construct. WT and Nuc1 astrocytes were transfected with these constructs and luciferase activity measured as readout for GFAP promoter activity ( Supplementary Fig. S7 ). WT astrocytes showed a much stronger GFAP promoter activity than did Nuc1 astrocytes. To test whether GFAP promoter activation is due to Notch signalling, we treated cells with DAPT before transfecting the cells with the promoter–reporter constructs. Both WT and Nuc1 astrocytes showed a reduction in GFAP reporter activity, confirming the role of the Notch pathway in differentiation of optic nerve astrocytes. The retina requires two macroglial cells, Muller cells and astrocytes, for proper functioning. While Muller cells are retina-specific, astrocytes are present throughout the central nervous system, and migrate from the optic nerve head into the inner retina [36] . Our studies with the Nuc1 spontaneous mutant rat, and the work of others, have demonstrated that in rodents an astrocyte template is essential for the proper formation of the retinal vasculature [24] , [37] , [38] , [39] . No signalling mechanisms have yet been shown to regulate formation of this template. Notch is the most significantly enriched signalling pathway in developing tissues and is known to regulate pattern formation in other systems; its dysfunction results in various developmental defects and adult pathologies [40] . We show that optic nerve astrocytes express both the Notch receptor and its ligand, Jagged1. This suggests that in astrocytes, Notch is involved in juxtacrine signalling, where Jagged1 from one astrocyte activates the Notch receptor on a neighbouring astrocyte. This juxtacrine signalling may be critical to the proper organization of astrocytes in the developing retina. In Nuc1, defective Notch signalling may account for improper template formation and patterning by retinal astrocytes. Notch signalling is known to have a pivotal role in cell fate specification during development. For example, it has been shown that blocking Notch signalling causes fewer Muller glial cells to be made in the retina, while an expansion of Muller glial cells was observed when Notch was activated [41] , [42] . Decreased Notch signalling in Nuc1 astrocytes may account for the abnormal morphology and decreased GFAP, which we have reported [24] , [43] . We now show lower gene promoter activity for GFAP in Nuc1 astrocytes, which might potentiate the decreased astrocyte number and abnormal template formation seen in the retinas of Nuc1 rats [24] , and in transgenic mice overexpressing the mutant βA3/A1-crystallin protein [43] . We have previously shown that in retinal-pigmented epithelial cells, βA3/A1-crystallin is trafficked to the lysosomes and has a pivotal role in the degradation of phagocytized photoreceptor outer segments [44] . This prompted us to investigate whether βA3/A1-crystallin modulates Notch signalling by manipulating lysosomal pH in astrocytes. Luminal acidification of endolysosomal compartments is regulated by a major proton pump, V-ATPase [45] . We show that βA3/A1-crystallin may affect endolysosomal acidification by regulating the activity of V-ATPase. Although organelles use the same V-ATPase to acidify their interiors, each is able to maintain a stable, characteristic internal pH [46] . V-ATPase activity is necessary for proper activation of Notch signalling in the endosomal system, although it is not required for Notch to access endosomal compartments [13] . In astrocytes, in which βA3/A1-crystallin is non-functional, the activity of V-ATPase is compromised, diminishing acidification of endolysosomal compartments and resulting in decreased Notch activation. This is consistent with studies showing that normal functioning of V-ATPase is required for optimal catalytic activity of γ-secretase [45] , [47] . Loss of functional βA3/A1-crystallin in astrocytes does not impede Notch ligand binding nor extracellular cleavages, because V-ATPase activity is only required after ligand binding. However, loss of βA3/A1-crystallin affects the γ-secretase-mediated processing of NICD in astrocytes. The resultant dysfunction, affecting release of NICD, inhibits transcription of Notch target genes. Lysosomes are cellular organelles primarily involved in degradation and recycling processes [48] . V-ATPase also has an important role in the lysosomal degradation of Notch [14] . Again, the regulation of proper luminal pH is critical for this process, as the lysosomal hydrolases that degrade internalized proteins, lipids and complex carbohydrates function optimally only in the acidified lysosomal microenvironment [15] . Our data on Cathepsin D, one such lysosomal hydrolase, is consistent with a general decrease in lysosomal hydrolase activity in astrocytes lacking βA3/A1-crystallin. In Nuc1 astrocytes, the Notch receptor does not undergo lysosome-mediated degradation at a normal rate, resulting in its abnormal accumulation. Similar results are seen in cells exposed to chloroquine, an inhibitor of lysosomal acidification [34] . As ligand-independent Notch activation does not normally occur in mammalian cells when Notch degradation is impaired [49] , acidification of the endolysosomal compartment in astrocytes is essential both for Notch signalling and degradation, suggesting a novel role for βA3/A1-crystallin as an important regulator of this acidification process. In conclusion, our study describes an unanticipated function for βA3/A1-crystallin in endolysosomal acidification in astrocytes as depicted in the hypothetical model ( Fig. 8i ). Regardless of the specific mechanism whereby mutation of βA3/A1-crystallin affects the activity of V-ATPase, and thus reduces endolysosomal acidification, our data suggest that through its action in maintaining normal lysosomal pH, βA3/A1-crystallin has a fundamental effect on Notch signalling in astrocytes. Antibodies The following antibodies were used: Notch1 (SAB3300078, Sigma, St. Louis, MO; ab27526, Abcam, Cambridge, MA; H731, Santa Cruz Biotechnology Inc., Santa Cruz, CA), Jagged1 (SC-8303, Santa Cruz Biotechnology Inc.), GFAP (Z0334, DAKO Corporation, Carpentaria, CA), Myc (2272S, Cell Signaling Technology, Danvers, MA), LAMP1 (H4A3-C, Developmental Studies Hybridoma Bank, University of Iowa, Iowa), Rab5 (C8B1, Cell Signaling Technology), Calnexin (ab75801, Abcam), Cathepsin D (SC-6487, Santa Cruz Biotechnology). Knockdown of βA3/A1-crystallin in astrocytes βA3/A1-crystallin ( Cryba1 ) floxed homozygous mice were generated. A BAC clone (Sp6 library, SV129 origin) encompassing the mouse βA3/A1-crystallin locus was obtained through the Invitrogen BAC screening service (Invitrogen, CA) and was used to construct a conditional targeting vector in which exons 4 and 5 were flanked by LoxP sites by recombineering as described [50] . The targeting vector contained a PGK-driven DTA (modified diphtheria toxin A) cassette [51] as the negative selection marker, and was electroporated into W4 (129S6/SVEvTac) ES cells [52] . G418-resistant clones were picked, expanded and screened for homologous recombination by both long-range genomic PCR and Southern blotting. Construction of the targeting vector containing the cKO allele was made as depicted in Supplementary Fig. 2 . Correctly targeted clones were further analysed by karyotyping. Embryonic stem cell clones carrying the targeted allele were isolated, and three clones were injected into blastocysts. The selectable marker (frt—Neo R —frt) was removed by mating to mice (Jackson Laboratories) expressing flp recombinase hACTB/FLPe (strain name: B6.Cg-Tg (ACTFLPe) 9205Dym/J) during early development. Successful excision of the selectable marker cassette was confirmed by PCR spanning the insertion site. Adenovirus infection Monolayer astrocytes from Cryba1 -floxed mice were infected with control adenovirus (Ad CMV eGFP) or Cre-recombinase virus (Ad CMV Cre-RSV GFP; KeraFAST Inc., Boston, MA). Ten thousand cells were infected in triplicate at MOI (multiplicity of infection) 0.01–10,000 p.f.u. per cell. Cell survival was assessed 48 h post infection by 3-(4,5-dimethylthiazol-2-yl)-2,5-diphenyltetrazolium bromide assay. Cells infected for 48 h were transfected with pcDNA3.1- Cryba1 vector to overexpress βA3/A1-crystallin and collected 36 h later. Primary culture of optic nerve astrocytes Optic nerve astrocytes from P2 rats (WT and Nuc1) and from P2 Cryba1- floxed mice were cultured in DMEM-F12 medium containing 10% fetal bovine serum, as recently described [53] . Quantitative reverse transcriptase PCR Two micrograms of total RNA was reverse-transcribed to cDNA in a 20-μl reaction volume using superscript reverse transcription kit (Invitrogen, Carlsbad, CA). PCR amplification was performed utilizing the 7500 PCR Fast Real-Time System (Applied Biosystems, Carlsbad, CA) with TaqMan probes for Notch1 (Rn01758633_m1), Notch2 (Rn01534371_m1), Jagged1 (Rn00569647_m1), Hey1 (Rn00468865_m1), Hes1 (Rn00577566_m1), NRP1 (Rn00686106_m1), HPRT(Rn01527840_m1) and GAPDH (Rn01775763_g1*). The reaction consisted of the following steps, enzyme activation at 95 °C for 20 s, 40 cycles of denaturation at 95 °C for 3 s combined with annealing/extension at 60 °C for 30 s. All data were analysed with the ABI 7500 real time PCR system using the data assist software (Applied Biosystems); graphs were plotted using Microsoft excel. All experiments were performed at least three times in triplicate. Data are represented as mean±s.d. Western blotting Western blots were done as previously described and quantified by densitometric analysis using ImageJ [54] . Luciferase assay For Notch luciferase assays, lipofectamine 2000 (Invitrogen) was used to transfect cells with the different Notch constructs and pGL2–6XCBF-1 Notch luciferase reporter construct (2.3 μg) together with pRL-SV40 (0.1 μg; Promega, Madison, WI) carrying the Renilla luciferase gene under the control of the cytomegalovirus promoter. Luciferase activity was measured using a luciferase assay system (Promega). The reporter activity was calculated by normalizing the firefly luciferase value with that of the Renilla luciferase control vector and expressed as relative luciferase units. All data were obtained from at least three independent experiments. The relative promoter activities were depicted as the mean±s.d. Immunofluorescence of cells and flat mounts Immunofluorescence was performed on cultured WT and Nuc1 cells, and retinal flat mounts as described [55] . Fluorescent images were taken with LSM 510 confocal microscope. siRNA treatment WT and Nuc1 astrocytes in 6-well plates were transfected with scrambled, Cryba1 or Jagged1 ON-TARGET plus SMARTpool siRNA (Dharmacon, Lafayette, CO). Plasmids The Notch expression plasmid NICD was generated by PCR from full-length Notch1 cDNA, corresponding to amino acids 1,760–2,556, and was cloned into pcDNA3.1 (Invitrogen). The NδE plasmid encodes the transmembrane and entire intracellular domain of murine Notch1, extending from I1701 to K2530 plus the C-terminal Myc tag in pcDNA3.1 mammalian expression vector (Invitrogen). The constructs NδE, NδE(V1744K) and ICv1744 were kindly provided by Dr Raphael Kopan and have been described [56] . Jagged1 overexpression plasmid containing a full-length rat Jagged1 was cloned into pCDNA3. Jagged1 EGF repeats were deleted using site-directed mutagenesis. Full-length rat Notch1 cDNA (Notch-FL), containing a single internal Myc epitope tag cloned into the pcDNA3.1. Notch extracellular truncation plasmid was made from the Notch-FL plasmid, and NICD plasmid was purchased from Addgene. A GFAP-promoter reporter vector containing 1.9 kb of the rat GFAP promoter upstream of the firefly cDNA was cloned into pGL2 vector as previously described [35] . Measurement of endolysosomal pH The luminal pH of endolysosomal vesicles was measured by a ratiometric method using a fluid-phase fluorescent marker, FITC-conjugated dextran (Invitrogen) [57] . Cells were incubated with FITC-dextran (500 μg ml −1 , Invitrogen) for 3 h to allow internalization of the fluorescent probe, then washed and resuspended in 50 mM MES buffer (pH 6.5), and the fluorescence measured at 520 nm by exciting at 450 nm and 495 nm. The fluorescence excitation ratio ( I 495nm / I 450nm ) was calculated, and endosomal pH determined from a calibration curve of FITC-dextran in the pH range of 4–7. To generate the calibration curve, cells loaded with FITC-dextran were collected and resuspended in 10 mM phosphate buffer supplemented with 2 mM FITC-dextran at 2 mg ml −1 and the measurements were made over time [58] . Lysosomal V-ATPase activity For the measurement of lysosomal V-ATPase activity, acridine orange uptake assay was performed with isolated lysosomes [59] . The lysosomes were suspended in buffer containing 6 μM acridine orange (Invitrogen), 150 mM KCl, 2 mM MgCl 2 and 10 mM Bis-Tris-propane. After a steady spectrofluorometric baseline was reached, V-ATPase was activated by addition of ATP (1.4 μM final concentration) and 2.5 μM valinomycin at pH 7.0 to promote the movement of K + from the inside to the outside of the lysosome, generating a membrane potential. Acridine orange uptake is a measure of V-ATPase-driven pumping of hydrogen ions into lysosomes. Fluorescence at 530 nm (excitation at 495 nm) was measured using a fluorescence plate reader (Bio-Tek Synergy, Winooski, VT). Separately, isolated lysosomes containing the same activation buffer were used to measure the extralysosomal quenching of acridine orange fluorescence. To confirm V-ATPase activity, stimulation of intralysosomal fluorescence and quenching of extralysosomal fluorescence were measured with or without 1 μM bafilomycin A1 (Sigma). Subcellular fractionations To prepare endosomal fractions, cells were homogenized in 1.5 ml of 2 M sucrose in HEPES-EDTA buffer containing protease and phosphatase inhibitor cocktails (Sigma). A PNS was prepared by centrifugation at 1,000 g at 4 °C for 10 min to remove the cell debris, followed by 3,000 g for 10 min to remove the nuclei. PNS (0.5 ml) was diluted 1:1 with sucrose (40%) and imidazole (3 mM) solution in HEPES-EDTA buffer. After overlay with 1.5 ml of 35% sucrose with 3 mM imidazole, 1 ml of 25% sucrose with 3 mM imidazole and 1 ml 8% sucrose with 3 mM imidazole, the sucrose gradients were centrifuged in a SW55 rotor (Beckman, Indianapolis, IN) at 150,000 g for 90 min. Translucent interfaces were collected from the top of the centrifuge tube. Cell homogenates were centrifuged at 3,000 g for 10 min to remove the nuclei and at 10,000 g for 15 min to remove the mitochondria. This supernatant was subjected to density gradient centrifugation and sample collection as described [32] . γ-Secretase activity assay The iodixanol fractions were incubated with 20 mM Hepes, 150 mM NaCl, 5 mM EDTA (pH 7.0), 0.4% CHAPSO and a protease inhibitor cocktail (Sigma) at 37 °C for 16 h with or without 1 μM of the γ-secretase inhibitor L-685,458 (Bachem, Torrance, CA). Reactions were stopped by addition of radioimmunoprecipitation assay buffer, heated to 95 °C for 5 min and centrifuged at 16,000 g for 5 min. Production of Aβ40 was analysed by ELISA with anti-Aβ40 antibody according to the manufacturer’s protocol (Wako chemicals, Richmond, VA). Production of Aβ40 was calculated as Aβ40 levels without L-685,458 minus Aβ40 levels with added L-685,458. Cells incubated with the lysosomal inhibitor, chloroquine, were also used to assay the activity of γ-secretase. Statistical analysis Statistical analysis was performed using Microsoft excel and GraphPad 5.0 software. The P -values were determined by two-tailed Student’s t -test in a triplicate experiment representative of at least three independent experiments. Multiple comparisons were made using Kruskal–Wallis test. Significance was defined as * P ≤0.05, * P ≤0.01. Results are presented as mean±s.d. Each biological replicate has at least five technical replicates. How to cite this article: Valapala, M. et al. Impaired endolysosomal function disrupts Notch signaling in optic nerve astrocytes. Nat. Commun. 4:1629 doi: 10.1038/ncomms2624 (2013).